Topological Fulde–Ferrell–Larkin–Ovchinnikov states in spin–orbit-coupled Fermi gases Pairing in an attractively interacting two-component Fermi gas in the absence of time-reversal symmetry or inversion symmetry may give rise to exotic superfluid states. Notable examples range from the Fulde–Ferrell–Larkin–Ovchinnikov state with a finite centre-of-mass momentum in a polarized Fermi gas to the topological superfluid (TSF) state in a two-dimensional (2D) Fermi gas under Rashba spin–orbit coupling and an out-of-plane Zeeman field. Here we show that a TSF state with a single-component nonzero centre-of-mass momentum, called a topological Fulde–Ferrell (tFF) state, can be stabilized in a 2D Fermi gas with Rashba spin–orbit coupling and both in-plane and out-of-plane Zeeman fields. The tFF state features a non-trivial Berry phase, along with unique properties that may be detected using existing experimental techniques. Since their original proposal in the 1906s, unconventional pairing states with finite centre-of-mass momentum have caught a considerable amount of attention in different physical contexts [1] , [2] , [3] , including organic superconductors [4] , heavy fermions [5] and dense quark matter [6] . Initially proposed as a compromise between superconductivity and finite magnetization, the key ingredient of this so-called Fulde–Ferrell–Larkin–Ovchinnikov (FFLO) state is a pairing mechanism between fermions having a finite centre-of-mass momentum. In the weak-coupling limit, this can be achieved by pairing particles residing either on distinct Fermi surfaces, as in the case of spin-polarized systems where spin-up and spin-down Fermi surfaces are mismatched, or on a single deformed Fermi surface which breaks the spatial inversion symmetry. The latter possibility has been discussed in the context of non-centrosymmetric superconductors, where spin–orbit coupling (SOC) of the Rashba ( σ x k x + σ y k y ) or the Dresselhaus type ( σ x k x − σ y k y ) would lead to a non-uniform superconducting state under external magnetic fields [7] , [8] , [9] , [10] , [11] . Here, σ i are the Pauli matrices and k i is the i th ( i = x , y , z ) component of the single-particle momentum. In ultracold Fermi gases, the pursuit of FFLO states has stimulated extensive investigation almost immediately after the realization of pairing superfluidity [12] . Recently, evidence for the FFLO superfluid has been reported in quasi-one-dimensional geometry at Rice Univeristy [13] . Meanwhile, the realization of synthetic SOC adds another important piece to the already versatile toolbox of controllability in cold atoms [14] , [15] , [16] , [17] . By Raman-coupling two hyperfine states in the ground state manifold of alkali atoms, experimentalists have implemented an equal mixture of Rashba and Dresselhaus SOC with both out-of-plane and in-plane effective Zeeman fields. In these experiments, the SOC strength depends on the wave vectors of the Raman lasers, and the effective out-of-plane (in-plane) Zeeman field is proportional to the Rabi frequency (two-photon detuning) of the Raman process. Theoretical investigation has demonstrated that the interplay of SOC, pairing superfluidity and effective Zeeman fields can lead to exotic superfluid phases in various dimensions [18] , [19] , [20] , [21] , [22] , [23] , [24] , [25] , [26] , [27] , [28] , [29] , [30] , [31] , [32] , [33] , [34] , [35] , [36] , [37] , [38] , [39] , [40] , [41] . In these systems, as SOC mixes different spin states, both intra- and inter-branch pairings can take place and the competition between them results in rich phase structures. An important example here is the topological superfluid (TSF) state in a two-dimensional (2D) Fermi gas with Rashba SOC and an out-of-plane Zeeman field [27] . The TSF state acquires a chiral Majorana edge mode protected by the gap in the bulk, and can be understood in the weak-coupling limit as a consequence of intra-branch pairing when the chemical potential lies within or below the gap opened by the out-of-plane Zeeman field. As both the inversion and the time-reversal symmetries are broken in the system, the TSF state belongs to class D. In this work, we show that a TSF state with a single-component nonzero centre-of-mass momentum, that is, a topological Fulde–Ferrell (tFF) state, can be stabilized in a 2D Fermi gas with Rashba SOC and both in-plane and out-of-plane Zeeman fields. Similar to the case of a TSF state, in the weak-coupling limit, the emergence of the tFF state can be understood as a result of single-branch pairing within the lower helicity branch. The application of the additional in-plane Zeeman field introduces deformation of the single-particle dispersion, and drives the system towards a more stable Fulde–Ferrell (FF) state. The resulting pairing state would preserve all topological properties provided that the deformation of the Fermi surface should not be drastic enough to violate the single-branch pairing scenario. This last condition is equivalent to the requirement that the introduction of the in-plane Zeeman field should not close the bulk gap. Thus, the topological nature of this state is protected by a full gap of quasi-particle spectra. This tFF state belongs to the same classification as that of the TSF state found in 2D Fermi gases with Rashba SOC [27] , and acquires all topological features including gapless edge states and Majorana zero modes in vortex cores [42] . We note that the centre-of-mass momentum of this tFF state is antiparallel to the in-plane Zeeman field. By mapping out the zero-temperature phase diagram, we further discuss the competition between various FF states with different centre-of-mass momentum. In particular, we find a nodal FF (nFF) state and characterize the evolution of its non-trivial gapless contours in momentum space. The tFF and nFF states should leave signatures in the species-selective momentum distribution and momentum-resolved radio-frequency spectroscopy, respectively, which, in principle, can be detected using existing experimental techniques. Phase diagram and the tFF state We consider a two-component Fermi gas in two dimensions with a Rashba SOC and both in-plane and out-of-plane Zeeman fields, where the Hamiltonian can be written as follows: Here, ξ k = ε k – μ , ε k = ħ 2 k 2 /2 m , a k σ ( ) is the annihilation (creation) operator for the pseudo-spin state σ with σ =(↑, ↓), m is the atomic mass, α denotes the strength of the SOC and HC stands for Hermitian conjugate. The out-of-plane ( h ) and in-plane ( h x ) Zeeman fields can be effectively induced depending on how the synthetic SOC is implemented. As an example, h and h x are proportional to the effective Rabi frequency and the two-photon detuning, respectively, of the Raman process in the current experimental scheme [15] , [16] . The bare s -wave interaction rate U should be renormalized as [43] : , where is the quantization area, and E b is the binding energy of the two-body bound state in two dimensions without SOC, which can be tuned, for instance, via the Feshbach resonance technique [44] . We focus on the zero-temperature properties of the system on the mean-field level, where the pairing order parameter , with Q the center-of-mass momentum of the pairing states. For pairing states with zero centre-of-mass momentum ( Q =0), analytical form of the dispersion spectrum can be obtained in the absence of the in-plane Zeeman field ( h x =0) [27] . In this case, a fully gapped TSF can be stabilized in a fairly large parameter region. The topological nature of this phase is characterized by a non-trivial topological number, and is protected by the underlying particle-hole symmetry. For the case of h x ≠0, it can be proved that the zero centre-of-mass momentum state becomes unstable against an FF state with pairing momentum . Thus, a topologically non-trivial FF state can be expected, provided that the in-plane field should not be large enough to close the gap of the bulk. To characterize the stability region of the tFF state, we map out the phase diagram on the plane of the SOC strength ( α ) and the chemical potential ( μ ), with fixed out-of-plane Zeeman field h and finite h x ( Fig. 1 ). Under the local density approximation, the phases traversed by a downward vertical line in the diagram represent those one should encounter by moving from a trap centre to its edge. From Fig. 1 , we see that the TSF phase in a 2D polarized Fermi gas with Rashba SOC and zero in-plane field is now replaced by a tFF phase with centre-of-mass momentum along the x -direction, as we have anticipated. 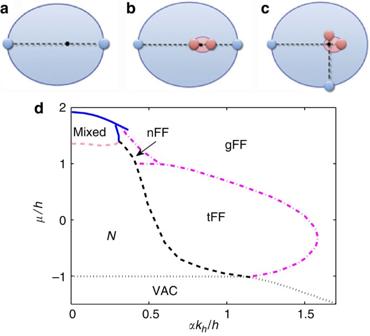Figure 1: Pairing mechanism and phase diagram. (a–c) Illustration of pairing mechanisms that give rise to different phases in the weak-coupling limit: (a) intra-branch pairing with a single Fermi surface, (b) intra-branch pairing with two Fermi surfaces and (c) inter-branch pairing. The filled areas with different colours represent the Fermi surfaces in the lower and upper helicity branches, and the black dot represents the origin of the momentum space. (d) Phase diagrams on theα−μplane forEb/h=0.5 andhx/h=0.1, whereEbis the binding energy of the two-body bound state in two dimensions without SOC. The solid curves are first-order boundaries, whereas the dash-dotted curves represent phase boundaries of continuous phase transitions. The dashed curves surrounding the normal region (N) are the threshold with ΔQ/h=10−3, whereas the dotted curves are the boundary against vacuum (VAC). In the weak-coupling limit, the tFF state corresponds to the pairing mechanism (a), the gapped FF (gFF) state and the nFF state correspond to the pairing mechanism (b), while (c) gives rise to a parameter region on the phase diagram where the global ground state is the result of competition between different FF states with centre-of-mass momentum in thex- or they-direction (mixed). The out-of-plane Zeeman fieldhis taken to be the unit of energy, whereas the unit of momentumkhis defined through. To characterize the non-trivial topological nature of this state, we further calculate the Berry phases associated with the two quasi-particle ( η =+, ν =1, 2) and two quasi-hole ( η =−, ν =1, 2) bands: Figure 1: Pairing mechanism and phase diagram. ( a – c ) Illustration of pairing mechanisms that give rise to different phases in the weak-coupling limit: ( a ) intra-branch pairing with a single Fermi surface, ( b ) intra-branch pairing with two Fermi surfaces and ( c ) inter-branch pairing. The filled areas with different colours represent the Fermi surfaces in the lower and upper helicity branches, and the black dot represents the origin of the momentum space. ( d ) Phase diagrams on the α − μ plane for E b / h =0.5 and h x / h =0.1, where E b is the binding energy of the two-body bound state in two dimensions without SOC. The solid curves are first-order boundaries, whereas the dash-dotted curves represent phase boundaries of continuous phase transitions. The dashed curves surrounding the normal region ( N ) are the threshold with Δ Q / h =10 −3 , whereas the dotted curves are the boundary against vacuum (VAC). In the weak-coupling limit, the tFF state corresponds to the pairing mechanism ( a ), the gapped FF (gFF) state and the nFF state correspond to the pairing mechanism ( b ), while ( c ) gives rise to a parameter region on the phase diagram where the global ground state is the result of competition between different FF states with centre-of-mass momentum in the x - or the y- direction (mixed). The out-of-plane Zeeman field h is taken to be the unit of energy, whereas the unit of momentum k h is defined through . Full size image where the Berry curvature is defined as [45] with the shorthand notation. The Berry phase of the superfluid state is then a summation over the contribution from the two occupied quasi-hole bands. A numerical evaluation shows that the resulting Berry phase vanishes in the topological trivial phase and becomes unity in the tFF state. As we have discussed before, the stabilization of the tFF state is due to the SOC-induced intra-branch pairing and the Fermi surface asymmetry. nFF states and topological phase transitions The simple picture of single-branch pairing becomes complicated with increasing chemical potential or increasing SOC intensity, such that particles on the higher helicity branch get involved into pairing. Due to the spin mixing induced by the SOC, both intra- and inter-branch pairings can take place with centre-of-mass momentum along either the x - or the y -direction. As a consequence, the ground state of the system is the result of competitions between the various FF pairing states, leading to a variety of FF states as depicted in Fig. 1 . In the case of strong SOC intensity, or equivalently weak out-of-plane Zeeman field, the ground state of the system becomes a topologically trivial FF state (gFF in Fig. 1 ), which is separated from the tFF state via a continuous phase boundary. This gFF phase is also fully gapped and with centre-of-mass momentum along the x axis. In the weak-coupling limit, the gFF phase corresponds to an intra-branch pairing in the presence of two Fermi surfaces. By tuning through the tFF–gFF phase boundary, the excitation gap closes and opens again, while the pairing order parameter Δ Q remains finite. A typical variation of the minimum excitation gap E g , the pairing order parameter Δ Q and the pairing momentum Q x with increasing chemical potential are plotted in Fig. 2a,b , respectively. 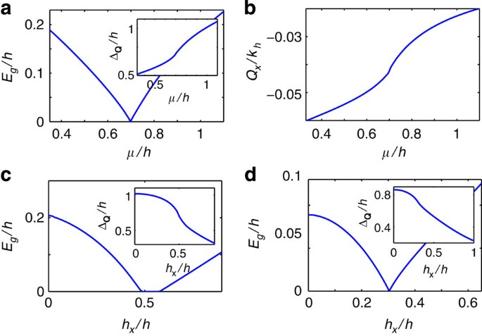Figure 2: Evolution of parameters across the topological phase boundary. (a,b) Evolution of the minimum excitation gap (a), the order parameter (a:inset) and pairing momentum (b) with increasing chemical potential. A full gap closes and opens again by traversing the continuous phase boundary between the tFF state and the gFF state. In these subplots,hx/h=0.1. (c,d) Evolution of the minimum excitation gap and the pairing order parameter (insets) with increasing in-plane fieldhx, with: (c)μ/h=1 and (d)μ/h=0.8. Other parameters used in this figure areEb/h=0.5 andαkh/h=1. Figure 2: Evolution of parameters across the topological phase boundary. ( a , b ) Evolution of the minimum excitation gap ( a ), the order parameter (a:inset) and pairing momentum ( b ) with increasing chemical potential. A full gap closes and opens again by traversing the continuous phase boundary between the tFF state and the gFF state. In these subplots, h x / h =0.1. ( c , d ) Evolution of the minimum excitation gap and the pairing order parameter (insets) with increasing in-plane field h x , with: ( c ) μ / h =1 and ( d ) μ / h =0.8. Other parameters used in this figure are E b / h =0.5 and αk h / h =1. Full size image Besides the gFF state, intra-branch pairing with two Fermi surfaces may also lead to an nFF phase. Indeed, close to the tFF and the gFF states, we identify a region on the phase diagram where the ground state is an nFF phase with pairing momentum along the x -direction, as depicted in Fig. 1 . This gapless superfluid state acquires two disconnected gapless contours in momentum space, which shrink to two separated gapless points and disappear at the continuous phase boundaries. A typical evolution of the two gapless contours are displayed in Fig. 3a with increasing chemical potential. In principle, these features can be reconstructed via momentum-resolved radio-frequency spectroscopy or Bragg spectroscopy. Notice that at the phase boundaries between the nFF and the gapped FF states (gFF or tFF), the quasi-particle and quasi-hole spectra touch the Fermi surface at different places (see Fig. 3c for example). This is in contrast to the phase boundary between the tFF and the gFF states, where the gap closes at a single point k =( Q x /2, 0) in momentum space (see Fig. 3d ). 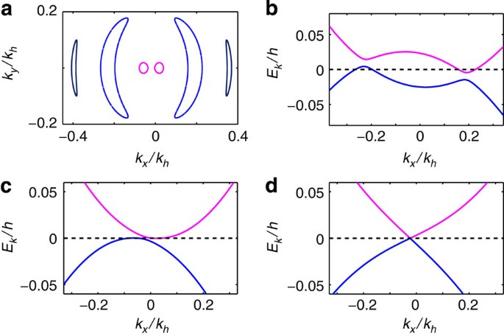Figure 3: Gapless contour and quasi-particle dispersion of the nFF state. (a) Evolution of gapless contours in the momentum space for the nFF states withαkh/h=0.49, andμ/h=1.002 (magenta), 1.05 (blue) and 1.15 (black). (b–d) Dispersion spectra of quasi-particle and quasi-hole along thekxaxis with (b)αkh/h=0.49,μ/h=1.05; (c)αkh/h=0.49,μ/h=1.002; and (d)αkh/h=0.8,μ/h=0.87. It is apparent from (c–d) that at the topological phase boundaries, two gapless points exist between the nFF and the tFF states, whereas a single gapless point exists between the gFF and the tFF states. Other parameters used in these plots areEb/h=0.5 andhx/h=0.1. Hence, the topological phase boundary between the tFF and the gFF states can be worked out by examining the gap closing condition Figure 3: Gapless contour and quasi-particle dispersion of the nFF state. ( a ) Evolution of gapless contours in the momentum space for the nFF states with αk h / h =0.49, and μ / h =1.002 (magenta), 1.05 (blue) and 1.15 (black). ( b – d ) Dispersion spectra of quasi-particle and quasi-hole along the k x axis with ( b ) αk h / h =0.49, μ / h =1.05; ( c ) αk h / h =0.49, μ / h =1.002; and ( d ) αk h / h =0.8, μ / h =0.87. It is apparent from ( c – d ) that at the topological phase boundaries, two gapless points exist between the nFF and the tFF states, whereas a single gapless point exists between the gFF and the tFF states. Other parameters used in these plots are E b / h =0.5 and h x / h =0.1. Full size image On the other hand, the topological phase boundary between the nFF and the tFF states needs to be determined numerically. Alternatively, the inter-branch pairing scenario can become significant with decreasing SOC intensity or increasing out-of-plane Zeeman field, which can effectively polarize the helices within each helicity branch and hence hinder intra-branch pairing. This gives rise to a parameter region on the phase diagram labelled as Mixed, where the global ground state is the result of competition between different FF states with centre-of-mass momentum in the x - or the y -direction. These states are typically very close in energy, and can be qualitatively understood as conventional FF states dressed by SOC. The phase transitions between the various FF states, the topological ones in particular, can also be investigated by sweeping the in-plane Zeeman field h x . In the weak-coupling limit, the presence of a larger h x shifts the upper helicity branch and enlarges the gap between two branches. As a consequence, the tFF state, which is dominated by the intra-branch pairing within the lower helicity branch, becomes stable in an extended parameter region, and the phase boundaries surrounding the tFF state are shifted towards larger values of chemical potential and SOC intensity. In Fig. 2c,d , we show the variation of the minimum excitation gap and the pairing order parameter with increasing in-plane field h x , indicating the two representative evolution paths of the system from gFF to nFF and eventually to tFF ( Fig. 2c ), or from gFF directly to tFF ( Fig. 2d ), depending on the starting point on the phase diagram. Finally, we note that although the various FF states discussed above acquire spatially modulating order parameters, we expect no supercurrent flow within the system. In fact, similar FFLO states under SOC have been investigated in the context of non-centrosymmetric superconductors, where explicit calculations in the weak-coupling limit gave zero supercurrent [10] , [11] . Momentum distribution across the topological phase boundary To characterize properties of the various phases on the phase diagram, we calculate their respective momentum distribution. In Fig. 4 , we show the momentum profiles of the minority spin component for cases within the tFF region (a and b) and the gFF region (c and d). It is apparent that the momentum distribution in a topologically non-trivial phase is drastically different from that in a topologically trivial phase. In particular, the density profile in momentum space for the minority spin features a dip in the tFF phase, in contrast to a peak in the gFF case. These results can be qualitatively understood by noticing that in the weakly interacting limit, the tFF state corresponds to intra-branch pairing within the lower helicity branch, where the population of the minority fermions is small around the point where the spin-mixing term vanishes. Meanwhile, the gFF state corresponds to the case of intra-branch pairing with two Fermi surfaces, where a filled upper helicity branch implies a maximally occupied minority spin state around the same location. 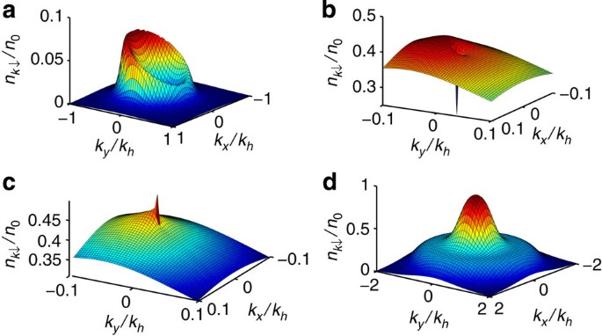Figure 4: Momentum-space density distribution for minority spin component. Parameters used in this plot are:Eb/h=0.5,hx/h=0.1,αkh/h=1,and the chemical potentials are: (a)μ/h=−0.85, (b)μ/h=0.6977,(c)μ/h=0.6980 and (d)μ/h=1. Notice that the momentum distribution features a dip for the tFF state (a,b), and a peak for the gFF state (c,d). Figure 4: Momentum-space density distribution for minority spin component. Parameters used in this plot are: E b / h =0.5, h x / h =0.1, αk h / h =1, and the chemical potentials are: ( a ) μ / h =−0.85, ( b ) μ / h =0.6977,( c ) μ / h =0.6980 and ( d ) μ / h =1. Notice that the momentum distribution features a dip for the tFF state ( a , b ), and a peak for the gFF state ( c , d ). Full size image The qualitative difference in momentum distribution of the minority fermions leads to an abrupt jump as the topological phase boundary is crossed. By extracting the momentum distribution from species-selective time-of-flight imaging, we may identify the tFF state in the underlying system. At present, only an equal mixture of Rashba and Dresselhaus SOC has been realized experimentally by Raman-coupling two hyperfine states in the ground state manifold of alkali atoms [14] , [15] , [16] . In these experiments, the effective Zeeman fields and the SOC strength are all dependent upon the laser parameters. This is also the case in most of the existing theoretical proposals for realizing Rashba SOC in ultracold atoms [46] , [47] . For instance, in ref. 47 , Liu et al . proposed to implement Rashba SOC in a 2D Fermi gas trapped in a lattice potential. Although the SOC there relies on periodically modulated Raman fields, the out-of-plane and the in-plane Zeeman fields can be realized and tuned by introducing two-photon detuning in the Raman processes, and on-site fields which couple the hyperfine spins, respectively. Experimentally, the relevant parameters are typically on the order of the recoil energy E r , which is estimated to be 2 πħ × 8.3 kHz in 40 K atoms [15] . For a Raman process consisting of counter-propagating lasers, a moderate Rabi frequency of 8 E r , and a small two-photon detuning of 0.8 E r should lead to the parameters h ~4 E r , h x ~0.4 E r and αk h / h ~1. For E b =0.5 h ~2 E r as chosen for Fig. 1 , the tFF state can be stabilized over a considerable range of the chemical potential. We stress that these parameters can be further optimized. At finite temperatures, we expect that the tFF state be stable below the Berezinskii–Kosterlitz–Thouless transition temperature, which is on the order of 0.1 T F for a 2D Fermi gas with SOC [28] , [30] . For a 2D Fermi gas without SOC, a temperature of T ~0.27 T F has recently been reported [48] . With these, it is reasonable to expect that the tFF state can be prepared and probed in future experiments. To summarize, we have investigated the pairing states of a 2D Fermi gas with Rashba SOC and both in-plane and out-of-plane Zeeman fields. Our results indicate the stabilization of a tFF state with centre-of-mass momentum antiparallel to the direction of the in-plane field. During the preparation of the final version of this article, we became aware of similar work by Qu et al., which also discusses the existence of a topological FFLO state in Fermi systems with spin-orbit coupling [49] . Mean-field formalism We focus on the zero-temperature properties of the FF pairing states with a single-valued centre-of-mass momentum on the mean-field level [1] , [2] . This should provide a qualitatively correct phase diagram at zero temperature. The effective mean field Hamiltonian can then be arranged into a matrix form in the hyperfine spin basis where Λ k = α ( k x + ik y )− h x and the order parameter . It is then straightforward to diagonalize the effective Hamiltonian and evaluate the thermodynamic potential at zero temperature where the quasi-particle ( η =+) and quasi-hole ( η =−) dispersions ( ν =1, 2) are the eigenvalues of the matrix in Hamiltonian (5), and Θ( x ) is the Heaviside step function. Without loss of generality, we assume h , h x >0, and Δ Q to be real throughout the work. The pairing order parameter Δ Q as well as the centre-of-mass momentum Q for the pairs can then be found by minimizing the thermodynamic potential in equation (6). Note that in general, the Hamiltonian (5) cannot be diagonalized analytically, and the thermodynamic potential needs to be evaluated numerically. Instability of the BCS state In the presence of a finite in-plane Zeeman field, the Fermi surface is deformed. In this case, the SOC-induced intra-branch pairing leads to the stabilization of an FF state with finite centre-of-mass momentum. The instability of Bardeen–Cooper–Schrieffer (BCS) pairing in this case can be checked by an expansion of the thermodynamic potential around the BCS pairing state with respect to small centre-of-mass momentum Q =( Q x , 0) where the expansion coefficients Ω i ( i =0,1,2 ⋯ ) can be evaluated numerically. We find that for finite h x , the second-order expansion coefficient Ω 2 is positive definite, whereas the first-order coefficient Ω 1 is always nonzero and has an opposite sign to that of h x . Hence, the ground state of the system under finite h x is an FF state with the centre-of-mass momentum antiparallel to the in-plane Zeeman field. This can be further checked by explicit evaluations of the thermodynamic potential (see Fig. 5 ). 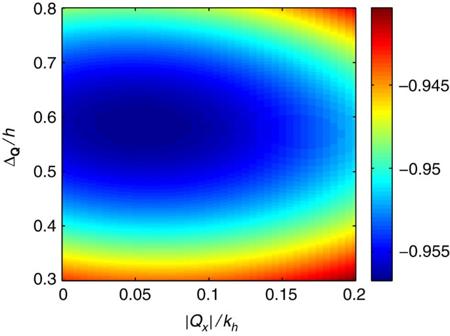Figure 5: Contour plot of thermodynamic potential. A typical case withEb/h=0.5,hx/h=0.1,αkh/h=1 andμ/h=0.5 is chosen to show the emergence of an FF state with finite order parameter ΔQand pairing momentum |Qx|. Figure 5: Contour plot of thermodynamic potential. A typical case with E b / h =0.5, h x / h =0.1, αk h / h =1 and μ / h =0.5 is chosen to show the emergence of an FF state with finite order parameter Δ Q and pairing momentum | Q x |. Full size image How to cite this article: Zhang, W. and Yi, W. Topological Fulde–Ferrell–Larkin–Ovchinnikov states in spin–orbit-coupled Fermi gases. Nat. Commun. 4:2711 doi: 10.1038/ncomms3711 (2013).